Two potential therapeutic antibodies bind to a peptide segment of membrane-bound IgE in different conformations IgE mediates hypersensitivity reactions responsible for most allergic diseases, which affect 20–40% of the population in developed countries. A 52-residue domain of membrane-bound IgE (mIgE) called CεmX is currently a target for developing therapeutic antibodies; however, its structure is unknown. Here we show that two antibodies with therapeutic potential in IgE-mediated allergic diseases, which can cause cytolytic effects on mIgE-expressing B lymphocytes and downregulate IgE production, target different conformations of an intrinsically disordered region (IDR) in the extracellular CεmX domain. We provide an important example of antibodies targeting an extracellular IDR of a receptor on the surface of intended target cells. We also provide fundamental structural characteristics unique to human mIgE, which may stimulate further studies to investigate whether other monoclonal antibodies (mAbs) targeting intrinsically disordered peptide segments or vaccine-like products targeting IDRs of a membrane protein can be developed. Omalizumab is a humanized mAb that binds to the CH3 domain of human IgE, near the binding site for the high-affinity type I IgE Fc receptors (FcεRI). It can neutralize free IgE and inhibit the IgE-mediated allergic pathway without sensitizing mast cells and basophils [1] , [2] . Omalizumab (trade name Xolair) has been shown in 60 completed clinical trials to be efficacious and safe for treating various IgE-mediated allergic diseases such as allergic asthma, allergic rhinitis and food allergy [3] , [4] , [5] , [6] as well as several non-allergic diseases that involve mast cells, such as chronic idiopathic urticaria [7] , [8] . Xolair has been approved in over 90 countries for treating patients with severe allergic asthma, uncontrollable even with high corticosteroid doses. These pharmaceutical developments have validated the IgE pathway as an effective therapeutic target for treating IgE-mediated allergic diseases [2] , [9] , [10] , [11] . The discovery of a 52-residue domain termed CεmX as part of the predominant isoform [12] of human membrane-bound ε chain (mε) ( Fig. 1a ) provides another approach to target the IgE pathway by reducing IgE production [2] , [12] . The gene segment encoding CεmX is only found in the mε of recently evolved primates, namely, the New-world monkeys and Old-world monkeys (including Homo sapiens ) [13] . CεmX is present in mε but not in membrane-bound immunoglobulin of other isotypes. To date, only two allelic forms differing by a leucine or valine at position 16 along the CεmX sequence (which generally does not affect antigenicity) have been found [14] . Although the three-dimensional (3D) structure of CεmX remains unsolved, previous work showed that two cysteines in CεmX form an intrachain disulfide bond (Cys-18 with Cys-39 or Cys-41), while the other two cysteines form an interchain bridge [15] . CεmX is thought to play a role in determining the outcome of cell signaling, following B cell receptor engagement [16] ; however, its function has not been fully elucidated. Unlike omalizumab that binds to both membrane-bound IgE (mIgE) and free IgE, an anti-CεmX antibody targets only mIgE and therefore can target mIgE-expressing B lymphoblasts and memory B cells to downregulate IgE production [17] , [18] without being neutralized by free IgE. Thus, a therapeutic anti-CεmX antibody could potentially be administered less frequently at smaller doses than omalizumab. 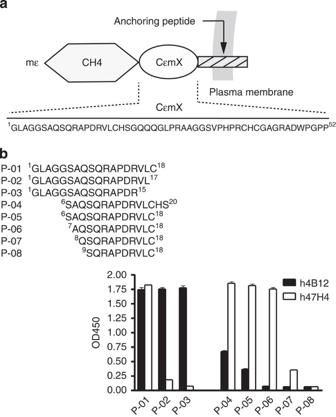Figure 1: Epitope mapping of anti-CεmX mAbs,h4B12andh47H4. (a) The CεmX sequence in human mIgE. (b) Reactivity of h4B12 and h47H4 with synthetic peptide segments of CεmX (P-01 to P-08). The mean and s.d. of triplicate measurements are shown. Figure 1: Epitope mapping of anti-CεmX mAbs, h4B12 and h47H4. ( a ) The CεmX sequence in human mIgE. ( b ) Reactivity of h4B12 and h47H4 with synthetic peptide segments of CεmX (P-01 to P-08). The mean and s.d. of triplicate measurements are shown. Full size image Here we analyse binding of two potential therapeutic humanized mAbs against human CεmX to their target. The antibody h4B12 from our group, derived from the parental murine mAb 4B12 (ref. 17 ), is in preparation to enter human clinical studies. The antibody h47H4 (quilizumab) from Genentech, derived from the parental murine mAb 47H4 (ref. 18 ), is in Phase IIb clinical trial for patients with moderate to severe allergic asthma. The 2.4-Å crystal structure of the complex of the Fab of h47H4 and a 35-residue CεmX peptide (PDB ID 3hr5) [18] shows that an 11-residue segment, 6 SAQSQRAPDRV 16 , is bound to h47H4, while the exact binding mode of h4B12 is not clear. In this work, we map the epitopes of these two potential therapeutic mAbs, determine the crystal structure of h4B12 Fab in complex with its peptide epitope, and present evidence that the dimeric CεmX domain is intrinsically disordered. Epitope mapping analysis of two anti-CεmX mAbs To define the epitopes of these two humanized mAbs, various CεmX peptides were synthesized and their affinities for h47H4 (which was prepared according to its published V H and V L sequences) and h4B12 were analysed using enzyme-linked immunosorbent assay (ELISA). Remarkably, the results show that h4B12 and h47H4 recognize overlapping, but different epitopes, and they do not crossreact with each other’s epitope. The first 15 CεmX residues ( 1 GLAGG SAQSQ RAPDR 15 ) bound h4B12 but not h47H4 ( Fig. 1b , P-03), whereas residues 7–18 ( 7 AQSQ RAPDR VLC 18 ) bound h47H4 but not h4B12 ( Fig. 1b , P-06). The results in Fig. 1b also indicate the CεmX residues that are critical for binding each of the two anti-CεmX mAbs. For h47H4, Cys-18 appears critical as its deletion nearly abolished binding to h47H4 but did not affect binding to h4B12 ( Fig. 1b , P-01 versus P-02). Ala-7 is also involved in discriminating the two mAbs, as its deletion dramatically reduced binding to h47H4 ( Fig. 1b , P-06 versus P-07). For h4B12, on the other hand, the first five CεmX residues, 1 GLAGG 5 , contributes to binding h4B12, as their deletion attenuates binding to h4B12 but not to h47H4 ( Fig. 1b , P-01 versus P-05). The next residue, Ser-6, also contributes to binding h4B12, as its deletion reduced binding to h4B12 but not to h47H4 ( Fig. 1b , P-05 versus P-06). Despite these differences, the two mAbs bind to a common 10-residue segment, 6 SAQSQ RAPDR 15 . The crystal structure of h4B12–peptide complex To determine how h4B12 binds to its epitope, we have determined the crystal structure of the h4B12 Fab in complex with its peptide epitope (excluding Gly-1), 2 LAGG SAQSQ RAPDR 15 at 1.92-Å resolution ( Fig. 2 and Table 1 ); Gly-1 was modeled into the 3D structure of the N-terminal CεmX using the PyMOL program [19] and energy-minimized to allow contact analysis of h4B12 Fab with its recognized full-length epitope, 1 GLAGG SAQSQ RAPDR 15 . The van der Waals and hydrogen-bonding interactions between h4B12 and its epitope shown in Fig. 3a appear consistent with the h4B12 ELISA results. The first five CεmX residues, 1 GLAGG 5 , bind h4B12 mainly via non-bonded contacts with Ile-56(H2), Gly-58(H2), Gly-91(L3), Val 94(L3) and Met-95(H3). The next CεmX residue, Ser-6, forms a backbone–backbone hydrogen bond with Gly-91(L3), while Gln-10 forms a sidechain–sidechain hydrogen bond with Asp-32(H1). The C-terminal 11 RAPDR 15 CεmX residues contact h4B12 through five hydrogen bonds with the L1, L2, H1 and H3 loops. 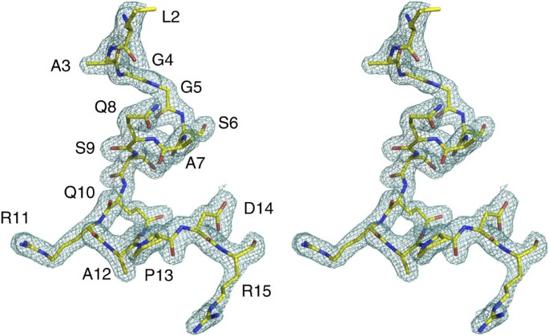Figure 2: The electron density map of the CεmX peptide bound byh4B12. 2LAGGSAQSQRAPDR15peptide was clearly defined in the 2Fo–Fcelectron density map contoured at 1.0 σ. Figure 2: The electron density map of the CεmX peptide bound by h4B12 . 2 LAGGSAQSQRAPDR 15 peptide was clearly defined in the 2 Fo–Fc electron density map contoured at 1.0 σ. Full size image Table 1 Data collection and refinement statistics. 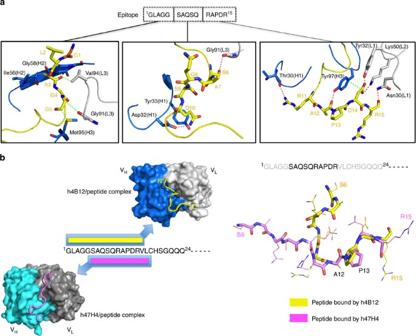Figure 3: The interaction between h4B12-Fab and its antigenic peptide and the conformations of the antigenic peptides when bound by h4B12 and h47H4. (a) The h4B12 Fab forms non-bonded contacts with1GLAGG5(left), two hydrogen bonds with6SAQSQ10(middle) and five hydrogen bonds with11RAPDR15(right). The CεmX peptide is in yellow with modeled Gly-1 in orange, the h4B12 VLis in grey and its VHis in blue. L and H denote complementarity-determining regions of VLand VH, respectively. Hydrogen bonds (red dashed lines) and van der Waals contacts (green dashed lines) are defined by a donor atom to an acceptor atom distance⩽3.5 and⩽4.0 Å, respectively. (b) The 1.9-Å structure of h4B12 FV(light grey and dark blue) and2LAGG SAQSQ RAPDR15(yellow) and the 2.4-Å structure of h47H4 (dark grey and light blue) and6SAQSQ RAPDRV16(violet) (left panel). Ala-12 and Pro-13 backbone nonhydrogen atoms in the common segment (6SAQSQRAPDR15) are superimposed to reveal the different peptide conformations in the two crystal structures (right panel). Full size table Figure 3: The interaction between h4B12-Fab and its antigenic peptide and the conformations of the antigenic peptides when bound by h4B12 and h47H4. ( a ) The h4B12 Fab forms non-bonded contacts with 1 GLAGG 5 (left), two hydrogen bonds with 6 SAQSQ 10 (middle) and five hydrogen bonds with 11 RAPDR 15 (right). The CεmX peptide is in yellow with modeled Gly-1 in orange, the h4B12 V L is in grey and its V H is in blue. L and H denote complementarity-determining regions of V L and V H , respectively. Hydrogen bonds (red dashed lines) and van der Waals contacts (green dashed lines) are defined by a donor atom to an acceptor atom distance ⩽ 3.5 and ⩽ 4.0 Å, respectively. ( b ) The 1.9-Å structure of h4B12 F V (light grey and dark blue) and 2 LAGG SAQSQ RAPDR 15 (yellow) and the 2.4-Å structure of h47H4 (dark grey and light blue) and 6 SAQSQ RAPDRV 16 (violet) (left panel). Ala-12 and Pro-13 backbone nonhydrogen atoms in the common segment ( 6 SAQSQRAPDR 15 ) are superimposed to reveal the different peptide conformations in the two crystal structures (right panel). Full size image Conformations of the peptides bound by h4B12 and h47H4 To determine the binding-mode differences between h4B12 and h47H4 to CεmX, we compared the peptide complex structure of h4B12 solved herein with that of h47H4 (PDB ID: 3hr5) [18] in Fig. 3b . The two mAbs bound the same peptide segment 6 SAQSQ RAPDR 15 in significantly different conformations, as shown in Fig. 3b . When the Ala-12 and Pro-13 backbone atoms of both peptides were superimposed, the ends of the two peptides diverged, as evidenced by a huge separation of 18.7 Å between the Ser-6 O γ atoms and 11.3 Å between the Arg-15 C ζ atoms. This disparity in the conformations of the two peptides bound by h4B12 and h47H4 suggests that this CεmX region may be intrinsically disordered. CεmX domain is intrinsically disordered To ascertain that CεmX contains intrinsically disordered region (IDRs), we employed various IDR algorithms to predict disorder in the entire CεmX domain [20] and measured the circular dichroism spectra of dimeric CεmX. Both approaches confirmed that CεmX contains IDRs. All the IDR algorithms [20] predict disorder for the first 12 CεmX residues ( Fig. 4a ). The meta–meta predictor GSmetaDisorderMD2 (ref. 20 ), which was the top-scoring method in the CASP9 benchmark, predicted the entire CεmX domain to be disordered. Notably, CεmX consists of 73% disorder-promoting residues (E, K, R, G, Q, S, P or A) and only 17% order-promoting ones (I, L, V, W, F, Y or C). In accord with the predictions, molecular dynamics simulations of the free peptides starting from their bound structures (PDB ID: 4lkx and 3hr5) show that both antigenic peptides do not adopt well-defined conformations in water (see Methods). Furthermore, the far UV circular dichroism spectra in Fig. 4b shows that dimeric CεmX, unlike ovalbumin, contains no signature profiles for ordered secondary structures (negative peaks at 208 and 222 nm for α helices and a negative peak at 217 nm for β sheets) but exhibits a negative peak at ~200 nm characteristic of a random coil. 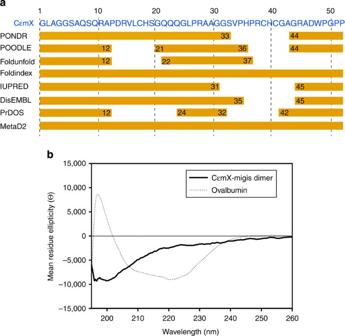Figure 4: Intrinsic disorder of the free CεmX peptide or domain. (a) Prediction of disorder (orange) in the CεmX domain by available servers. (b) Far UV circular dichroism spectra of dimeric CεmX and the migis-ε domain (black curve) and ovalbumin (dotted grey curve). Figure 4: Intrinsic disorder of the free CεmX peptide or domain. ( a ) Prediction of disorder (orange) in the CεmX domain by available servers. ( b ) Far UV circular dichroism spectra of dimeric CεmX and the migis-ε domain (black curve) and ovalbumin (dotted grey curve). Full size image Previous studies have shown that IDR-containing proteins exist broadly in all life forms and play crucial roles in recognition, regulation, cell signaling and control pathways [21] , [22] , [23] , [24] , and IDRs are prevalent in disease-associated proteins such as p53, c-Myc transcription factor, α-synuclein and glycogen synthase kinase 3β [24] , [25] , [26] . Since IDRs often interact with multiple partners with high specificity but low affinity [22] , [27] , they are considered as drug targets for small molecules that interfere with the binding of these IDRs to their binding partners [28] . Indeed, small drug-like molecules that block the binding of an IDR in p53 to murine double minute 2 have been developed and the drug candidates such as MI-219 and Nutlin-3 are undergoing Phase I clinical trial for the treatment of retinoblastoma cancer [29] . In addition, several antibodies targeting disordered loop regions of disease-associated proteins such as viral protein hemagglutinin [30] have been reported. However, no study had shown that antibody drug molecules can target an extracellular IDR of a receptor on the surface of a targeted cell type with the desired cytolytic effects. This study shows that potential therapeutic antibodies targeting IDRs of a protein drug target may be prepared. An advantageous feature of an IDR is its ability to adopt different structures upon binding to different partners. In analogy to the C-terminal IDR of p53 that is involved in ‘one-to-many’ binding [31] , the N-terminal IDR of CεmX can adopt a twisted-coil or an extended-coil conformation upon binding to h4B12 or h47H4, respectively. The fact that a region of a protein exists in an intrinsically disordered state does not preclude the generation of antibodies binding to this region with high affinity and high specificity. Antibodies generated by immunization of a peptide segment of a protein can bind to the free peptide segment with high affinity. Although some anti-peptide antibodies do crossreact with comparable affinity with the native proteins when the peptide is flexible within the native structure—for example, antibodies against peptide segments of hemagglutinin [32] and lysozyme [33] —they generally bind to the denatured protein [34] . In contrast, h4B12 and h47H4 bind to the same CεmX peptide segment of native mIgE in quite different conformations with high affinity and specificity. Furthermore, they cause the lysis of mIgE-expressing B cells, thus downregulating IgE production [17] , [18] . Notably, h47H4 has advanced to phase IIb clinical trial. Both h4B12 and h47H4 can bind to mIgE on B lymphocytes and mediate cytolytic mechanisms on mIgE-expressing B cells through apoptosis and antibody-dependent cellular cytotoxicity [17] , [18] . The antigenic sites for those two mAbs are not blocked by possible CεmX-binding partner(s) or by associated molecules on the cell surface. This is important since not all regions of CεmX are accessible to mAbs [17] . The IDR algorithms ( Fig. 4a ) predicted that the C-terminal CεmX segment of about 10 residues is also intrinsically disordered. Earlier work showed that mAbs could bind strongly to this peptide segment in CεmX-containing proteins in a cell-free system [35] , but not to mIgE on B lymphocytes. This suggests that the terminal segment of CεmX is blocked by adjacent molecules on the cell surface [17] or by possible CεmX-binding partner(s). This study suggests a novel way to elucidate intrinsic disorder by inducing a disordered region to adopt different structures upon binding to different mAbs and determining the mAb-bound structures using X-ray crystallography, NMR or other spectroscopic methods. It has provided the first structural characterization of the entire dimerized CεmX region ( Fig. 4b ), which is not only an important drug target, but also is unique in that CεmX is found solely in mIgE but not in free IgE or other immunoglobulin classes. The significance of an intrinsically disordered CεmX domain is that more than one specific, high-affinity antibody can be developed to target CεmX in native mIgE and cause cytolytic mechanisms. It prompts investigations as to whether CεmX or its IDRs could be used to prepare vaccine-like products for use in patients to elicit antibody response against CεmX and hence downregulate the mIgE-expressing B cells. Hence, this work should encourage the development of therapeutic antibodies that bind with high specificity and affinity to extracellular IDRs in other drug target proteins. The findings herein highlight the difference between the two isoforms of mIgE found in humans. If the asymmetric sIgE structure were to apply to mIgE (whose structure is unknown), mIgE would require a substantial conformational change to enable the Fab regions to bind antigen [11] . Our results suggest that the highly flexible, disordered CεmX region of mIgE enables such a conformational change, allowing the Fab regions to reorient and bind antigen. Thus, compared with the non-CεmX-containing mIgE, the additional flexibility provided by the long-form mIgE has advantages for binding antigen, possibly accounting for its dominance over its short-form counterpart [12] . ELISA binding assays Peptides used for epitope mapping were synthesized at the Peptide Core Laboratory of the Genomics Research Center in Academia Sinica, Taiwan. The ultra pure peptides used for crystallization were synthesized by Genomics Inc. (Taipei, Taiwan) and dissolved in 10 mM Tris buffer stock solution at a concentration of 30 mg ml −1 . For epitope mapping, peptides of 10 μg ml −1 were coated on wells of a 96-well plate at 4 °C overnight. After blocking with 1% bovine serum albumin, 1 μg ml −1 of h4B12 or h47H4 was added to the wells. The plate was then incubated at room temperature for 2 h, and horseradish peroxidase-conjugated goat anti-human IgG diluted 1:20,000 was added to the wells. After incubating for 1 h at room temperature, the signal was developed by TMB solution and the absorbance at OD 450 was measured. IgG1 Fc·CεmX+migis and h4B12 Fab expression and purification The IgG1 Fc·CεmX+migis (migis is the extracellular portion of the C-terminal transmembrane peptide segment) and h4B12 Fab proteins were expressed in FreeStyle 293F suspension culture cell expression system and medium (Invitrogen, CA). Transfection of targeted genes into 293F cells was performed at a cell density of 10 7 cells ml −1 in 600-ml culture in 2-L Erlenmeyer flasks using linear polyethylenimine with an average molecular weight of 25 kDa (Polysciences, Warrington, PA) as a transfection reagent. The transfected cells were incubated at 37 °C for 4 h in an orbital shaker (125 r.p.m. ), and their cell density was then adjusted to 2.5 × 10 6 cells ml −1 with fresh medium and incubated for 4–5 days. Culture supernatants were harvested, and IgG1 Fc·CεmX+migis and h4B12 Fab in the media were purified using Protein A and KappaSelect chromatography, respectively. Crystallization and X-ray structure determination The h4B12-Fab (44 mg ml −1 ) and the CεmX peptide 2 LAGSAQSQ RAPDR 15 (10 mg ml −1 ) were mixed and subjected to crystallization trials using the hanging-drop vapour diffusion method with a protein-to-reservoir ratio of 1 μl:1 μl. From the initial crystallization screening, crystals of h4B12 complexed with the peptide were obtained using a reservoir containing 0.1 M sodium acetate trihydrate at pH 4.6, 25% PEG4000 and 0.2 M ammonium sulfate. The crystals were grown at 16 °C and the reservoir volume was 500 μl. They were soaked for 5 s in the reservoir solution containing 25% (v/v) glycerol as a cryoprotectant. X-ray data were collected at a wavelength of 0.97622 Å on beamline BL13C1 at NSRRC in Hsinchu, Taiwan using the MAR300 CCD detector. All data were processed and integrated using the programs Denzo and Scalepack in the HKL2000 suite [36] (see Table 1 ). Calculation of Matthews coefficient suggested that the asymmetric unit contains one protein molecule. The h4B12-Fab structure was solved by molecular replacement with the Phaser Program [37] using the light chain of the Fab structure (PDB ID: 3AAZ) and the heavy chain of the Fab structure (PDB ID: 2JIX) separately as a search model. The programs Coot [38] , PHENIX [39] and REFMAC5 (ref. 40 ) were used in model building and refinement, while the sigma A-weighted 2 F o– F c electron density map guided the model-building process. In the complex structure, most of the h4B12 Fab structure was modeled into the good 2 Fo – Fc map; the electron density for residues Ser-127–Thr-131 of the heavy chain was not visible. Unambiguous electron density of Ala-3–Asp-14 of the bound peptide was seen at 2.5-σ cutoff in the initial Fo – Fc difference map. Among these residues, the electron density maps for the side chain of Ser-6, Gln-10 and Pro-13 were most defined; therefore, the model of the bound peptide was built using these three residues as the base. The complex structure was improved by rigid-body, positional and restrained refinement with individual isotropic B-factors using PHENIX [39] and REFMAC5 (ref. 40 ). The statistics of the final model are listed in Table 1 . Molecular dynamics simulations The 14-residue 2 LAGGSAQSQRAPDR 15 and 11-residue 6 SAQSQRAPDRV 16 peptides were extracted from their X-ray structures complexed with h4B12 (this work) and h47H4 (3h5r), respectively, and were subjected to 16 ns molecular dynamics simulations using the CHARMM [41] version 37 program and the CHARMM27 all-atom parameter set [42] . All Asp residues were deprotonated, whereas Arg residues were protonated. The resulting peptide with a net charge of +1 was neutralized by adding a chloride counterion at the position of highest electropositivity with the constraint that the counterion was ≥7 Å from the peptide surface. The neutral system was solvated in a truncated octahedron containing TIP3P water molecules [43] , resulting in a total of 15,209 or 15,191 atoms. To relieve any bad contacts in the solvated peptide structure, the water molecules were subjected to rounds of minimization with constraints on the protein heavy atoms. The resulting solvated system was subjected to molecular dynamics at a mean temperature of 300 K using a 2 fs timestep, periodic boundary conditions, van der Waals interactions shifted to zero at 12 Å and electrostatic interactions treated via the particle mesh Ewald summation method [44] . Initially, 40 ps of dynamics was performed with the peptide backbone atoms and counterions restrained by a harmonic potential, which was then removed for the rest of the 16 ns simulation where the coordinates were saved every 2 ps. The saved 7,500 conformations were clustered pairwise using the Maxcluster program [45] , which computes the root-mean-squared deviations of the C α atoms and clusters conformations that are within 2.5 Å of the cluster centroid. For the 14-residue 2 LAGGSAQSQRAPDR 15 peptide, 99.5% of the 7,500 saved conformations could be grouped into 47 clusters with the largest three clusters accounting for only 35% of the sampled conformations, whereas for the 11-residue 6 SAQSQRAPDRV 16 peptide, 99.8% of the conformations could be assigned to 17 clusters with the top three clusters accounting for 73% of the sampled conformations. Disorder predictions The CεmX sequence was submitted to the following publicly available intrinsic disorder predictors: PONDR VL-XT [46] ( pondr.com/index.html ), POODLE-S [47] ( http://mbs.cbrc.jp/poodle/poodle-s.html ), FoldUnfold [48] ( http://skuld.protres.ru/~mlobanov/ogu/ogu.cgi ), Foldindex [49] ( http://bip.weizmann.ac.il/fldbin/findex ), IUPRED [50] ( http://iupred.enzim.hu , using short algorithms), PrDOS [51] ( http://prdos.hgc.jp/cgi-bin/top.cgi ), DisEMBL [52] ( http://dis.embl.de ) and MetaDisorderMD2 (MetaD2) [20] ( http://iimcb.genesilico.pl/metadisorder/ ). We used the default parameters in each algorithm and refer the reader to the cited references for details of each method. Digestion and purification of dimeric CεmX-migis proteins The IgG1.Fc-CεmX-migis fusion protein was incubated with recombinant enterokinase (rEK) to remove the dimeric CεmX-migis regions and nonCεmX residues, Gly and Ser at the N-terminus. The rEK and the fusion protein at a ratio of 1:50 (unit μg −1 ) were incubated at 25 °C overnight. rEK was removed using EKapture Agarose (Novagen) according to the manufacturer’s instructions. The mixture without rEK was applied to a Protein A column to remove the IgG1 Fc and incompletely digested material. The dimeric CεmX-migis was collected in the flow-through; EKapture Agarose was again added to remove any rEK contaminant and buffer-exchanged into PBS buffer using a PD-10 column. Circular dichroism spectra Circular dichroism spectra were monitored on a Jasco 815 dichrograph using 1-mm-thick quartz cells in 10 mM sodium phosphate buffer, pH 7.4, at 20 °C. They were measured between 195 and 260 nm, with a scanning speed of 20 nm min and a data pitch of 0.1 nm. Spectra were averaged from three scans and smoothed using the ‘means-movement’ smoothing procedure implemented in the SpectraManager package. The contribution of buffer was subtracted from experimental spectra. Mean ellipticity values per residue ([Θ]) were calculated as [Θ]=3,300 m ΔA/( l c n ) in degrees cm 2 dmol –1 , where m is the molecular mass in Daltons, ΔA is differential absorbance of left and right circularly polarized light, l is the path length equal to 0.1 cm, c is the protein concentration equal to 0.1 mg ml −1 and n is the number of residues, which is 138 for dimeric CεmX-migis. Accession code. The atomic coordinates reported in this paper have been deposited in Protein Data Bank with accession code 4LKX . How to cite this article: Chu, H.-M. et al. Two potential therapeutic antibodies bind to a peptide segment of membrane-bound IgE in different conformations. Nat. Commun. 5:3139 doi: 10.1038/ncomms4139 (2014).